Imaging Coulomb islands in a quantum Hall interferometer In the quantum Hall regime, near integer filling factors, electrons should only be transmitted through spatially separated edge states. However, in mesoscopic systems, electronic transmission turns out to be more complex, giving rise to a large spectrum of magnetoresistance oscillations. To explain these observations, recent models put forward the theory that, as edge states come close to each other, electrons can hop between counterpropagating edge channels, or tunnel through Coulomb islands. Here, we use scanning gate microscopy to demonstrate the presence of QH Coulomb islands, and reveal the spatial structure of transport inside a QH interferometer. Locations of electron islands are found by modulating the tunnelling between edge states and confined electron orbits. Tuning the magnetic field, we unveil a continuous evolution of active electron islands. This allows to decrypt the complexity of high-magnetic-field magnetoresistance oscillations, and opens the way to further local-scale manipulations of QH localized states. The quantum nature of electrons is two-sided: discreteness of charge and wave-like behaviour. Most of the time, experiments reveal either one or the other. Quantum rings (QRs) are known to be archetype devices in which the wave-like nature of electrons manifests itself through Aharonov–Bohm (AB) oscillations [1] . They originate from the magnetic field B -dependence of the phase acquired by electrons along the arms of the QR, which modulates electron interferences within the QR. Therefore, in the coherent regime of transport and at low B , the resistance of a mesoscopic QR exhibits oscillations as B is varied, with a flux period corresponding to the flux quantum [2] ϕ 0 = h/e . On the other hand, charge quantization can dramatically affect transport through a nanoscopic island occupied by N electrons. When the charging energy is e 2 / C >> k B T , where C is the island capacitance and T is the temperature, Coulomb blockade (CB) prohibits electron transport, except for potential values, such that N and N +1 states are degenerated [3] . CB manifests itself by periodic conductance peaks when the electrostatic potential is varied. In contrast, in the QH regime, the situation should be simpler: resistance vanishes at low temperature as transport occurs through edge states [4] , [5] , [6] . Several local probe experiments have confirmed this edge-state picture and imaged localized states in the bulk of macroscopic two-dimensional electron systems [7] , [8] , [9] , [10] . However, numerous experiments on mesoscopic devices in the QH regime revealed surprising observations, such as pseudo-AB 'subperiods' and 'superperiods' [11] , [12] , [13] , [14] , [15] , [16] , [17] . Motivated by these unexpected results, recent theories brought to the fore the discrete nature of electrons to explain the broad range of periodicities. They invoke Coulomb interactions and tunnelling between an electron island and edge states [18] ( Fig. 1 ), which may be combined with a spatial oscillation of the outermost electron orbit in the island [17] . Complementing these theories, simulations yielded a detailed microscopic description of the different possible processes taking place in this regime [19] , [20] . To the theoretical debate is added the diversity of experimental observations, which hampers unambiguous determination of the precise mechanisms at the local scale. 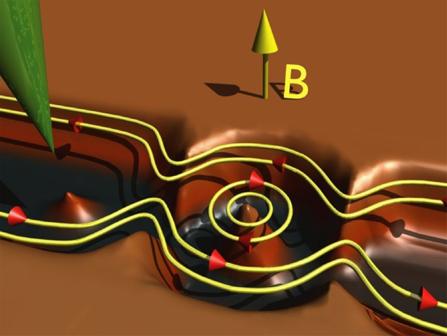Figure 1: An artist's view of edge states in the quantum ring confining potential. To simplify, we have assumed that no edge state is reflected at the ring's openings, which may not be the case in the real quantum ring. The tip (in green) induces a local perturbation of the potential that can be scanned over the quantum Hall interferometer. Figure 1: An artist's view of edge states in the quantum ring confining potential. To simplify, we have assumed that no edge state is reflected at the ring's openings, which may not be the case in the real quantum ring. The tip (in green) induces a local perturbation of the potential that can be scanned over the quantum Hall interferometer. Full size image Here, we present a spatially resolved investigation of electron transport inside an interferometer formed by an InGaAs/InAlAs QR (see Methods), driven in the integer QH regime. We show that each pseudo-AB period can be associated with a specific Coulomb island formed by edge state loops enclosing a hill or a valley in the potential. Each active Coulomb island can be located precisely inside the QR by tuning the magnetic field and imaging the spatial shift of Coulomb resonances by means of scanning gate microscopy (SGM). Magnetoresistance measurements At low B and T , electron transport through the QR is in the coherent regime. This is attested by periodic AB oscillations in resistance R versus B . As expected, the AB period Δ B AB =9 mT ( Fig. 2c ) corresponds to the average QR radius (380 nm). Note also that the QR is in the quasi-ballistic regime (the electron mean free path is ~800 nm at low B ), and ~25 transverse modes are transmitted through the QR's openings (the Fermi wavelength is 22 nm, and the width of the openings is 250 nm). At high B , the two-dimensional electron system enters into the QH regime and its transverse magnetoresistance R xy versus B exhibits plateaus at values h /( νe 2 ), where ν is the (integer) filling factor ( Fig. 2a ). Within the plateaus, the Hall bar longitudinal magnetoresistance R xx versus B drops to zero. In contrast, in the B -range coinciding with the position of the plateaus, the magnetoresistance of QR shows strong reproducible fluctuations with a wide range of characteristic B -scales ( Fig. 2b–f ). In Fig. 2b , we also note the absence of finite resistance plateaus, which would indicate a difference in the number of filled Landau levels (LLs) in the bulk and in the constrictions [15] . A closer look at R versus B in the region near ν =6 reveals high-frequency periodic oscillations over some parts of the high B -range ( Fig. 2f ), with a period Δ B =1.5 mT that is much smaller than that of the AB oscillations. 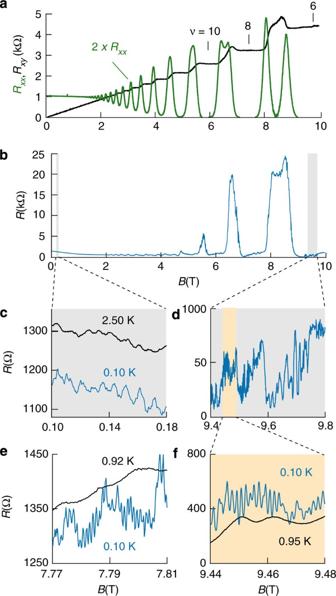Figure 2: Magnetoresistance measurements on the Hall bar and on the quantum ring. (a) Longitudinal and transverse (Hall) resistancesRxxandRxyversusB, measured in the Hall bar. Overshoots inRxyoriginate from a mixing of longitudinal and Hall resistances, due to a geometrical asymmetry of the Hall bar. (b) Magnetoresistance of the quantum ring (QR). (c) Low-Bmagnetoresistance of the QR, measured atT=0.1 and 2.5 K. The periodicity of oscillations inRversusBis ΔB=9 mT. (d) Magnetoresistance of the QR on the quantum Hall (QH) plateau aroundν=6, atT=0.1 K. (e) Magnetoresistance of the QR on the QH plateau aroundν=8,T=0.1 and 0.92 K. The periodicity of the oscillations inRversusBis ΔB=1.1 mT. (f) Close-up of (d) in the orange-shaded region, atT=0.1 and 0.95 K. The periodicity of the oscillations inRversusBis ΔB=1.5 mT. Figure 2e shows that a similar pattern is also visible on the plateau near ν =8, but with an even shorter period, Δ B =1.1 mT. Finally, these high- B oscillations decay rapidly with temperature ( Fig. 2e,f ) and vanish before reaching 1 K. This contrasts with AB oscillations that, similar to the phase coherence time, saturate below ~1 K [21] and are still visible at 2.5 K ( Fig. 2c ). An alternative mechanism, which is unrelated to electron interferences, must therefore be invoked to explain our observations. Figure 2: Magnetoresistance measurements on the Hall bar and on the quantum ring. ( a ) Longitudinal and transverse (Hall) resistances R xx and R xy versus B , measured in the Hall bar. Overshoots in R xy originate from a mixing of longitudinal and Hall resistances, due to a geometrical asymmetry of the Hall bar. ( b ) Magnetoresistance of the quantum ring (QR). ( c ) Low- B magnetoresistance of the QR, measured at T =0.1 and 2.5 K. The periodicity of oscillations in R versus B is Δ B =9 mT. ( d ) Magnetoresistance of the QR on the quantum Hall (QH) plateau around ν =6, at T =0.1 K. ( e ) Magnetoresistance of the QR on the QH plateau around ν =8, T =0.1 and 0.92 K. The periodicity of the oscillations in R versus B is Δ B =1.1 mT. ( f ) Close-up of ( d ) in the orange-shaded region, at T =0.1 and 0.95 K. The periodicity of the oscillations in R versus B is Δ B =1.5 mT. Full size image To explain the presence of subperiod oscillations, a recent theory invokes CB of electrons tunnelling between the conducting edge states transmitted along the borders of the QR and those forming a QH electron island located at the centre of the device [18] ( Fig. 1 ). Changing the magnetic field redistributes electrons within the LLs: if the flux through the area A enclosing the island increases by one flux quantum ϕ 0 , one electron must be added to each filled LL. This process introduces a new contribution to the island charging energy, with a magnetic field period ΔB =( φ 0 / A )/ f c = ΔB AB / f c , where f c is indeed the number of filled LLs. In turn, charging energy oscillations affect the QR resistance through the CB of electrons tunnelling between the QH island and the transmitted edge states. Note that the area encircled by edge states at high B is not necessarily equal to the mean area A of the QR, which determines Δ B AB . Simulations (not shown here) of the electron local density of states at B =9.5 T in a 2DEG with the same Fermi energy as in the experiment indicate that the outermost populated edge state extends 55 nm away from the edge of the device. Taking this value and edge roughness into account, an edge state loop encircling the central QR antidot would therefore have a radius that is similar to the QR mean radius. This explains the remarkable consistency between the prediction of pseudo-AB subperiods Δ B AB / f c and our observations that Δ B =1.5 and 1.1 mT around ν =6 and 8, respectively ( Fig. 2e,f ). From the analysis of QR magnetoresistance oscillations, a QH Coulomb island should therefore be present in our QR. Although our sample geometry is a priori well suited to generate a quantum island around the central antidot, it could, as we will see later, locate elsewhere. Therefore, local-scale information is needed to strengthen our understanding. In addition, the observation of subperiod oscillations only in narrow B -windows remains to be explained. Scanning gate microscopy Combining electron transport measurements with local probe techniques has already proven to be powerful in the investigation of the local details of electron behaviour inside various mesoscopic systems such as quantum point contacts [22] , [23] , [24] , open and closed quantum dots [25] , [26] , [27] , and quantum interferometers in the AB regime [28] , [29] , [30] , [31] . The technique, namely SGM, consists of scanning the electrically biased tip of an atomic force microscope (AFM) in a plane parallel to the 2DES and recording the changes in QR resistance R ( x , y ), which is induced by the tip located at ( x , y ). In the context of the experiments conducted in this study, the intrinsic sensitivity of CB to potential variations makes SGM potentially well suited to explore Coulomb islands. In the B -range in which subperiod oscillations were evidenced, the resistance map R ( x , y ) reveals a first set of concentric fringes (type I) centred on the QR antidot ( Fig. 3a ). Qualitatively, this is exactly the behaviour expected for a gate scanning above an electron island experiencing CB, that is, fringes correspond to isopotential lines located at uniform distances from the island [26] , [27] . It is worth noting that it is indeed the flux through the edge state loop that controls the present CB effect. Hence, it can be tuned either by sweeping B or by approaching a negatively polarized tip that raises the potential and enlarges the loop surface. Each concentric type-I fringe in Fig. 3a can therefore also be viewed as an isoflux line that marks one single CB state. Note that the observed succession of concentric fringes is reminiscent of patterns evidenced in previous SGM experiments on a QR at low B [28] , but the physical origin is totally different. As they vanish with increasing T , type-I fringes leave a more apparent second set of fringes (type II), which is found T -independent below 1 K ( Fig. 3b,c ). The presence of two distinct phenomena is made even clearer in Fig. 3d , representing the T -dependence of δ R , the standard deviation of R ( x , y ) in the rectangular regions labelled A and B in Fig. 3c , which mainly encompass type-I and type-II fringes, respectively. 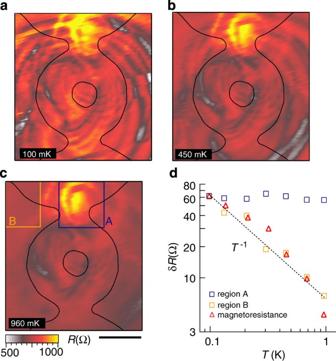Figure 3: Scanning gate resistance maps of the quantum ring (QR), showing Coulomb island-related concentric rings. (a–c)R(x,y) map obtained atB=9.5 T,Vtip=−1 V and atT=100, 450 and 960 mK, respectively. The black curves correspond to the position of the QR. The scale bar represents 500 nm. (d)T-dependence of δR, calculated on rawR(x,y) maps in regions A and B defined in (c) (blue and orange squares, respectively) and on high-pass filteredRversusBtraces (red triangles). The frequency of the high-pass filter onRversusBcurves is 60 T−1, and δRin this case is evaluated in the range of 9.47–9.53 T. Figure 3: Scanning gate resistance maps of the quantum ring (QR), showing Coulomb island-related concentric rings. ( a – c ) R ( x , y ) map obtained at B =9.5 T, V tip =−1 V and at T =100, 450 and 960 mK, respectively. The black curves correspond to the position of the QR. The scale bar represents 500 nm. ( d ) T -dependence of δ R , calculated on raw R ( x , y ) maps in regions A and B defined in ( c ) (blue and orange squares, respectively) and on high-pass filtered R versus B traces (red triangles). The frequency of the high-pass filter on R versus B curves is 60 T −1 , and δ R in this case is evaluated in the range of 9.47–9.53 T. Full size image Focusing on type-I fringes, we note that they exhibit the same T- dependence as the subperiod oscillations in the magnetoresistance ( Fig. 3d ). More precisely, the T −1 -dependence of δ R is compatible with a CB origin for both observations. Indeed, in classical CB experiments at B =0 T, the conductance peak height was reported to scale as δ G T −1 in the case of single-level transport through a lateral quantum dot [3] , [32] . In our case, electrons transmitted through Coulomb islands contribute only to a part of the total conductance (δ G/G ≈δ R/R <0.1). Therefore, δ R and δ G should effectively exhibit the same T- dependence. Different frameworks can be invoked to explain the origin of type-II fringes. First, in the QH regime, potential variations are at the origin of 'hot spots', that is, regions of high sensitivity of resistance to local potential changes, which have been evidenced by SGM in a Hall bar at 1.9 K [33] . This may explain type-II patterns observed within the area of the QR . But the concentric ring-like patterns at the QR opening (region A, Fig. 3c ) cannot be explained within this model, as 'hot spots' do not give rise to an oscillatory behaviour in resistance when the tip approaches the spot. As an alternative, we suggest that the tip can modulate tunnelling processes between counterpropagating edge states [18] at the openings. Affecting more than one edge state with the tip potential would induce the observed concentric pattern. Magnetoresistance measurements could confirm this scenario: indeed, R versus B should exhibit finite resistance plateaus in the case of a tip-induced difference in the number of filled LLs inside the QR and at the openings [15] . Up to now, we have analysed only a small B -range in which ΔB AB / f c subperiods dominate. A close look at Fig. 2d reveals that changing the magnetic field by only a few percents (for example, from 9.5 to 9.7 T) strongly modifies the magnetoresistance. This time, marked AB-like 'superperiod' oscillations show up, with Δ B =17 mT ( Fig. 4a ), which share the same T −1 -dependence (not shown) as the subperiods discussed above. According to the Rosenow–Halperin model [18] , superperiod oscillations indicate much smaller edge state loops. With an enclosed area A =( φ 0 / ΔB )/ f c =4×10 −14 m 2 , the loop should have a mean radius of ~65 nm, and hence be located somewhere in the arms of the 300-nm-wide QR. Our scanning gate should therefore be able to locate the loop. 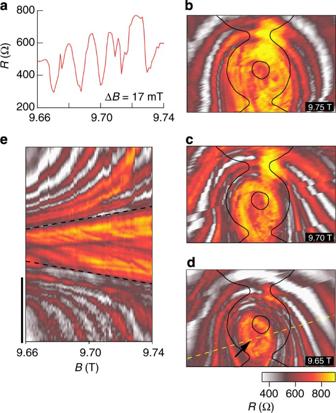Figure 4: Changing the magnetic field reveals the position of a Coulomb island on scanning gate microscopy maps. (a)RversusBatT=100 mK. (b–d)R(x,y) maps obtained atB=9.75, 9.70 and 9.65 T, respectively, withT=100 mK andVtip=−1 V. (e)B-dependence of theR(x,y) profile measured along the dashed line in (d). The vertical scale bar represents 1 μm. Figure 4: Changing the magnetic field reveals the position of a Coulomb island on scanning gate microscopy maps. ( a ) R versus B at T =100 mK. ( b – d ) R ( x , y ) maps obtained at B =9.75, 9.70 and 9.65 T, respectively, with T =100 mK and V tip =−1 V. ( e ) B -dependence of the R ( x , y ) profile measured along the dashed line in ( d ). The vertical scale bar represents 1 μm. Full size image The SGM localization is achieved in the sequence shown in Figure 4b–d . From 9.75 to 9.65 T, fringes shrink and finally reveal the active Coulomb island, indicated by the arrow in Fig. 4b . Note that the precise shape of the central SGM pattern is a convolution of the Coulomb island and the tip's potential shape [34] . A more detailed view of this process is shown in Fig. 4e , displaying the B -dependence of the SGM profile taken along the dashed line in Fig. 4d , crossing the centre of the fringes. Clearly, isoresistance lines shift towards lower B as the negatively charged tip approaches. Interestingly, the sign of the B -shift can indeed discriminate between edge states surrounding a potential hill and those confined to the border of the potential well. Assuming that the incompressible island surrounds a potential hill, approaching a negative-biased tip will raise the potential and increase the loop surface. If the incompressible island were localized in a potential well, the tip would reduce the loop surface. As isoresistance lines correspond to isoflux states through the incompressible loop, the low- B shift in Fig. 4e unambiguously identifies the fact that the loop surrounds a potential hill. It is worth noting that both subperiods and superperiods are observed in limited B -ranges. This means that a small potential perturbation by the tip could completely wipe out CB oscillations, by either suppressing tunnelling channels or suppressing CB islands. The region delimited by the dashed lines in Fig. 4e provides an example of such a state in which AB-like superperiods are suppressed. 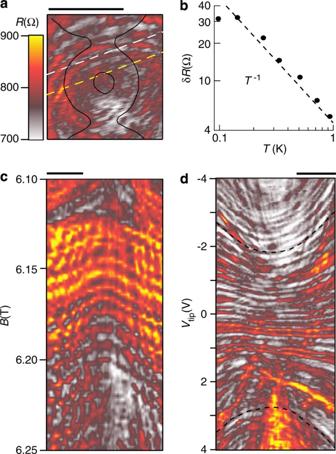Figure 5: Shift of Coulomb blockade resonances with magnetic field and tip voltage. (a)R(x,y) map measured atB=6.25 T andVtip=−0.5 V. (b)T-dependence of δRmeasured from anR(x,y) map atB=6.25 T. (c)B-dependence of theR(x,y) profile measured along the yellow dashed line in (a). (d)Vtip-dependence of theR(x,y) profile measured along the white dashed line in (a). The black line at the top of each graph represents 1 μm. At first sight, the data taken near ν =10 and shown in Figure 5a resemble more SGM maps presented in another QR but at low B [28] . Strikingly, the B -dependence of the profile taken along the yellow dashed line in Fig. 5a shows dominant oscillations with Δ B ~7.8 mT ( Fig. 5c ), which is very close to what the orthodox AB effect would provide in our sample. However, the temperature dependence, shown in Figure 5b , is not that expected for the AB effect. Indeed, the observed resistance oscillations are only pseudo-AB ones, as they exhibit the same T −1 -dependence as the sub- and superperiod oscillations, indicating that they share the same CB origin. Figure 5: Shift of Coulomb blockade resonances with magnetic field and tip voltage. ( a ) R ( x , y ) map measured at B =6.25 T and V tip =−0.5 V. ( b ) T -dependence of δ R measured from an R ( x , y ) map at B =6.25 T. ( c ) B -dependence of the R ( x , y ) profile measured along the yellow dashed line in ( a ). ( d ) V tip -dependence of the R ( x , y ) profile measured along the white dashed line in ( a ). The black line at the top of each graph represents 1 μm. Full size image As already shown near ν =6, CB resonances shift towards low B when the tip approaches the QR ( Fig. 5c ). However, the relative amplitude of this shift is smaller compared with that shown in Figure 4e , because the tip does not scan directly over the active Coulomb island; therefore, the potential perturbation experienced by the Coulomb island is not as large as that shown in Figure 4e . In addition, the data reveal a much richer pattern of fringes, indicating that multiple Coulomb islands are at work. This is confirmed in Fig. 5d , which shows the V tip -dependence of SGM profiles taken along the white dashed line in Fig. 5a (note that changing the position of the SGM profile yields qualitatively similar results). The main features are parabolic-like iso-resistance lines, indicated by the dashed lines. Their curvature evolves from zero at V tip =0 V to positive or negative, according to the polarity of the tip, as expected for Coulomb interaction between the tip and a potential hill (see also ref. 27 ). However, similar to Fig. 5c , Fig. 5d also shows steeper resistance lines, confirming the richness and complexity of mesoscopic transport in QH interferometers. The wealth of behaviour exhibited in SGM data at different magnetic fields and tip voltages illustrates the capability of SGM to embrace the complexity of QH interferometers at the local scale, and, beyond that, of mesoscopic transport. The fine-tuning of the local-scale potential by the biased tip offers various opportunities to image and manipulate localized electron states. Such a detailed probing of electron transport in QH interferometers may also prove to be valuable in future explorations of non-abelian quantum states [35] , [36] . Device fabrication and sample parameters The QR was patterned using electron beam lithography and wet etching in an InGaAs/InAlAs heterostructure [37] . A two-dimensional electron system is confined 25 nm below the surface and its low-temperature electron density and mobility are 1.4×10 16 m −2 and 4 m 2 /V s, respectively, as calculated from longitudinal and transverse magnetoresistance ( R xx and R xy versus B , Fig. 2a ) measurements on a Hall bar patterned next to the QR. The inner and outer lithographic radii of the QR are 215 and 520 nm, respectively, and the width of both openings is 300 nm ( Supplementary Fig. S2 ). Note that the depletion length at the edge of etched trenches is ~25 nm. SGM technique The experiments are carried out down to 100 mK, with the sample thermally anchored to the mixing chamber of a 3 He/ 4 He dilution refrigerator, and a home-made AFM suspended underneath. The force sensor consists of a commercial AFM cantilever coated with 20 nm of Ti and 10 nm of Pt (model CSC17 from MikroMasch; nominal tip radius: 40 nm), glued on one prong of a quartz tuning fork using conductive silver epoxy ( Supplementary Fig. S1a ). To measure the sample topography, the AFM is operated in the dynamic mode with a feedback loop on the tuning fork oscillation frequency shift. Using this method, we obtained the topography image of the QR shown in Supplementary Figure S2a , at a temperature T =100 mK. Clear edges are visible where the heterostructure was etched, which is an indication of a sharp tip. Further information on the quality of both the tip and the imaging technique can be inferred by comparing the topography image ( Supplementary Fig. S2a ) with Supplementary Fig. S2b , obtained by scanning electron microscopy (SEM) before cooling down the sample. Small differences can be observed between Supplementary Fig. S2a and b . In particular, the size of the etched trenches is ~100 nm smaller in the AFM topography. This discrepancy originates from the convolution of the tip shape with the surface topography in the AFM picture. Supplementary Fig. S1b shows an image of the extremity of the tip used in the experiments presented in this work, which is obtained by SEM after the end of the SGM experiments. The size of the tip apex in this picture is ~70 nm, which explains the difference in dimensions between Supplementary Fig. S2a and b . After imaging the topography of the ring, the tip is lifted at a distance of ~50 nm from the sample surface (that is, 75 nm away from the 2D electron system), and a bias voltage V tip is applied to the tip to induce a local electrostatic perturbation for electrons transmitted through the QR. QR resistance R is measured using a low-frequency (28 Hz) lock-in technique, with the source-drain voltage across the QR always being less than k B T / e . Figures 4b–d were measured over several hours. Before and after such a set of SGM experiments, the QR topography was imaged to check whether the tip drifted with respect to the QR position during the experiment. We observed that the lateral drift was always smaller than 50 nm. An additional shift between the topography and the R ( x , y ) map may originate from differences between the topographic tip and the 'electric tip', that is, the perturbation of electrostatic potential associated with the charged tip, experienced by electrons inside the QR. Indeed, charged contamination on both the tip and the sample surface may contribute to alter this potential. This shift can be roughly estimated by noting that each set of concentric resistance fringes in R ( x , y ) maps is centred on a Coulomb island, and must therefore have its centre located within the limits of the QR. By examining all the available R ( x , y ) maps, we could determine a higher bound of ~150 nm on this shift (that is, a shift larger than 150 nm would mean that some sets of resistance fringes are centred outside the QR area). A crucial issue in the context of SGM is the 'gating behaviour' of the tip [34] , [38] . First, Supplementary Fig. S1b shows that the metal layer covering the tip apex remained continuous during our experiment, and was not damaged by the numerous topographic scans realized at low temperature. In addition, there is no indication of a multiple tip in Supplementary Fig. S1b , topography mode or in SGM images. Complementarily, the electrical quality of the tip can be evaluated from the R ( x , y ) maps. In the R ( x , y ) map shown in Supplementary Figure S3 , neighbouring resistance fringes separated by less than ~50 nm can be distinguished, which gives an indication of the width of the perturbating potential. Note that this width increases with the tip-surface separation in SGM mode. Furthermore, the electrical potential associated with the charged tip should ideally have a circular symmetry to avoid unwanted distortion of the features visible in the R ( x , y ) map. This symmetry can be evaluated on SGM maps of quantum dots: when the tip potential shifts an energy level of the quantum dot in resonance with the source and drain energy levels, electrons can tunnel through the quantum dot, which induces a current rise. In an SGM map, these resonances are visible as sets of concentric rings. The set of rings is directly related to the electrical potential of the tip, as shown in ref. 34 . In our experiment, the sets of resistance fringes in R ( x , y ) maps are also related to the CB phenomenon and correspond to isopotential lines. Their precise shape depends both on the tip potential shape and on the shape of the potential hill around which each electron loop is localized. In the case of an anisotropic tip potential, the sets of resistance fringes in R ( x , y ) maps would all exhibit the same shape distortion related to the potential anisotropy. This is contrary to our observations: we observe a large diversity in the shapes of resistance fringes, but no recurrent anisotropy. This indicates that the tip potential shape is not anisotropic. How to cite this article: Hackens, B. et al . Imaging Coulomb islands in a quantum Hall interferometer. Nat. Commun. 1:39 doi: 10.1038/ncomms1038 (2010).